GANP regulates recruitment of AID to immunoglobulin variable regions by modulating transcription and nucleosome occupancy Somatic hypermutation in B cells is initiated by activation-induced cytidine deaminase-catalyzed C→U deamination at immunoglobulin variable regions. Here we investigate the role of the germinal centre-associated nuclear protein (GANP) in enhancing the access of activation-induced cytidine deaminase (AID) to immunoglobulin variable regions. We show that the nuclear export factor GANP is involved in chromatin modification at rearranged immunoglobulin variable loci, and its activity requires a histone acetyltransferase domain. GANP interacts with the transcription stalling protein Spt5 and facilitates RNA Pol-II recruitment to immunoglobulin variable regions. Germinal centre B cells from ganp -transgenic mice showed a higher AID occupancy at the immunoglobulin variable region, whereas B cells from conditional ganp -knockout mice exhibit a lower AID accessibility. These findings suggest that GANP-mediated chromatin modification promotes transcription complex recruitment and positioning at immunoglobulin variable loci to favour AID targeting. Affinity-maturation of antibodies, which takes place in antigen (Ag)-driven B cells at germinal centres (GCs) of peripheral lymphoid organs is achieved through generation of somatic hypermutation (SHM) at immunoglobulin (Ig) variable (V)-region genes [1] , [2] , [3] , [4] . SHM depends on activation-induced cytidine deaminase (AID), which is specifically upregulated in GC B cells. AID initiates SHM by catalyzing C→U conversion at the rearranged Immunoglobulin variable (IgV)-locus as the initial step of SHM [1] , [2] , [3] , [4] and class switch recombination [5] . AID is predominantly localized in the cytoplasm in activated B cells [6] but is targeted preferentially to Ig genes in the nucleus through interaction with its recruiting partners. Interacting proteins that have been suggested in various assays to form a complex with AID include single-stranded (ss) DNA binding protein RPA (ref. 7 ), kinases DNA-PKcs (ref. 8 ) and Protein Kinase A (refs 9 , 10 ), adaptor protein 14-3-3 (ref. 11 ); a group of proteins involved in transcription and mRNA processing, CTNNBL1 (ref. 12 ), PTBP2 (ref. 13 ), SRSF1 (ref. 14 ), RNA exosome subunits [15] , Spt5 (ref. 16 ), Spt6 (ref. 17 ), RNA polymerase II (Pol-II) [18] , RNA Pol-II associated factor 1 (PAF1) complex [19] , and others such as EXPO1/Crm1 (ref. 20 ), Hsp90 (ref. 21 ), Hsp40 DnaJa1 (ref. 22 ), MDM2 (ref. 23 ), eEF1A (refs 17 , 24 ), REGγ (ref. 25 ), KAP1/Trim28 (refs 17 , 26 ) and HP1 (ref. 26 ). Germinal centre-associated nuclear protein (GANP) associates with AID in the cytoplasm and facilitates its recruitment to the nucleus, eventually enhancing AID access to actively transcribed IgV-loci [27] . GANP expression is ubiquitous in mammalian cells but is increased in Ag-driven GC B cells [28] . B cells from GANP -deficient mice failed to generate high levels SHM at the rearranged IgV-locus and could not generate affinity-maturation of Ag-specific antibodies [29] . Reciprocally, transgenic overexpression of GANP increased the frequency of high-affinity Ab-producing cells against immunized Ags in vivo [30] . Thus, GANP is critical in generation of high-affinity antibodies in GC B cells during immune responses [31] . GANP is a 210-kDa nuclear protein with multiple domains having different functions. A domain in the middle portion of GANP is homologous to the Saccharomyces Sac3 (refs 32 , 33 ). Sac3 is a component of transcription-export complex 2 (TREX-2), a ribonucleoprotein (RNP) complex involved in mRNA export in yeast [34] . Besides the Sac3-homology domain, the N-terminal region of GANP is homologous to FG/SP-rich nucleoporin (Nup) proteins [32] , [35] . GANP carries a putative RNA recognition motif situated between the Nup domain and Sac-homology domain, and its C-terminus contains a histone-acetyltransferase (HAT) domain that regulates minichromosome maintenance protein 3 (MCM3) [36] . An alternatively spliced variant of GANP mRNA was reported in humans. A shorter isoform of GANP, GANP/MCM3AP (ref. 37 ), is likely to encode an 80-kDa protein associated with MCM3 of the DNA helicase MCM-complex composed of MCM2-MCM7 (refs 28 , 38 ) and possesses HAT activity. Based on the Sac3-homology domain, GANP has been shown to play important roles in the mRNA export of mammalian cells [35] , [39] . However, the overall function of mammalian GANP has not been determined. In particular, the detailed molecular mechanism describing how GANP regulates SHM at the IgV-locus has largely remained unclear. Here, we analyse GANP-interacting proteins in B cell nuclei by a proteomics strategy and study the function of GANP in the regulation of chromatin organization and interaction with the RNA Pol-II transcription complex at the IgV-region. Our data show that GANP is involved in histone modification and interaction with transcription elongation factors at the IgV-region, and that this allows for AID recruitment to IgV-loci during SHM in B cells. GANP-interacted proteins in hypermutating B cell nuclei We performed a proteomics screen for GANP-interacting proteins in Ramos B cells that constitutively undergo a low level of SHM (ref. 40 ). Proteins extracted from nuclei were co-immunoprecipitated (IP) with two different GANP antibodies and were subjected to analysis by two-dimensional image-converted analyses of liquid chromatography and mass spectrometry (2DICAL) [41] , [42] (see Supplementary Fig. S1a ). By comparing about 5,000 peptide peaks in anti-GANP co-IP precipitates to IgG co-IP control ( Supplementary Fig. S1b ), we identified over 100 peptide peaks present at significantly higher levels ( P- value <0.05) in GANP co-IP precipitates. The largest proportion of the peptides belongs to histones (28%), followed by proteins involved in RNA splicing/processing proteins (22%), ribosomal proteins (16%), nuclear envelope proteins (11%), RNA/DNA helicases (7%), chromatin regulators (4%), and DNA-dependent kinases (3%) ( Fig. 1a and Supplementary Table S1 and S2 ). GANP interactions with several helicases DHX9, DDX21 and DDX39, nuclear envelope proteins Nups, DNA-PKcs, and DNA topoisomerase 2a were confirmed by co-IP assays ( Supplementary Fig. S2 ). 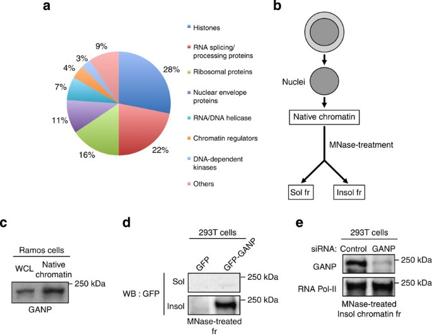Figure 1: GANP interacts with histones and associates with chromatin. (a) GANP-associated proteins in Ramos cells. 2DICAL analysis was used to identify about 100 proteins co-immunoprecipitated with GANP, but not with IgG control. The proteins are classified according to their biological functions. (b) Schematic representation of chromatin fractionation using MNase. (c) Western blot (WB) analysis of GANP in chromatin fractions prepared from Ramos cells. Whole-cell lysate (WCL) is shown for control. (d) WB analysis of 293 T cells transfected with a GFP-GANP expression vector. Soluble (Sol) and insoluble (Insol) chromatin fractions were isolated by digesting native chromatin with MNase. Each fraction was blotted with anti-GFP Ab. (e) 293 T cells were transfected with Control or GANP siRNA and harvested after 3 days. The insoluble chromatin fraction was prepared and blotted with anti-GANP (upper) and anti-RNA Pol-II (lower) antibodies. Data in (c–e) are from one of three sets of independent experiments with similar results. Figure 1: GANP interacts with histones and associates with chromatin. ( a ) GANP-associated proteins in Ramos cells. 2DICAL analysis was used to identify about 100 proteins co-immunoprecipitated with GANP, but not with IgG control. The proteins are classified according to their biological functions. ( b ) Schematic representation of chromatin fractionation using MNase. ( c ) Western blot (WB) analysis of GANP in chromatin fractions prepared from Ramos cells. Whole-cell lysate (WCL) is shown for control. ( d ) WB analysis of 293 T cells transfected with a GFP-GANP expression vector. Soluble (Sol) and insoluble (Insol) chromatin fractions were isolated by digesting native chromatin with MNase. Each fraction was blotted with anti-GFP Ab. ( e ) 293 T cells were transfected with Control or GANP siRNA and harvested after 3 days. The insoluble chromatin fraction was prepared and blotted with anti-GANP (upper) and anti-RNA Pol-II (lower) antibodies. Data in ( c – e ) are from one of three sets of independent experiments with similar results. Full size image Given the interaction of GANP with histones, we examined whether GANP is associated with chromatin in the nucleus. Nuclear protein extracts were subjected to differential chromatin fractionation using micrococcal nuclease (MNase) ( Fig. 1b ). Chromatin binding was confirmed for endogenous GANP in Ramos B cells ( Fig. 1c ). 293 T cells were transfected with GFP-GANP and used for chromatin fractionation. GFP-GANP was observed only in the insoluble (Insol) chromatin fraction but not in the soluble (Sol) chromatin-free fraction. Tight binding to chromatin was confirmed for GANP in 293 T cells ( Fig. 1d ) and verified by a GANP knockdown experiment ( Fig. 1e ). GANP knockdown led to a significant decrease in the level of GANP in the chromatin fraction, whereas the level of chromatin-associated RNA Pol-II control protein was not affected. Together, the data suggest that GANP interacts with histones and associates tightly with chromatin. GANP affects assembly of nucleosomes at the IgV-regions The C-terminus of GANP contains a domain with a high similarity to HAT ( Fig. 2a ) [36] , [43] . We examined whether the HAT domain of GANP (HAT G ) possesses histone acetylation activity and plays a role in B cells. First, a recombinant HAT G tagged with the glutathione S -transferase at the N-terminus (GST-HAT G ) was expressed and purified from E. coli and incubated with histone H3 or H1 in the presence of acetyl-coenzyme A ( Fig. 2a ). Time dependent acetylation of histones H3 and H1 was observed in the presence of GST-HAT G , but not GST-control, indicating that the HAT G domain has histone acetylation activity ( Fig. 2a ). 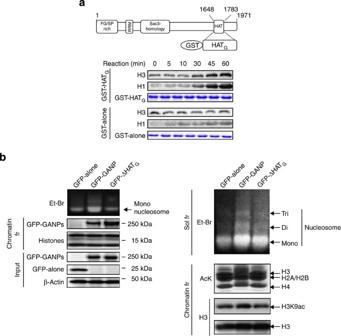Figure 2: The histone acetylation activity of GANP modulates chromatin assembly and nucleosome organization. (a) The HAT domain of GANP (HATG) possesses histone acetylation activity. Recombinant GST-HATGor GST-alone protein (100 ng) was incubated with histone H3 or H1 (1 μg) in the presence of acetyl-coenzyme A (10 μM). Acetylated histones H1 and H3 were analysed by WB. (b) MNase sensitivity assay for Ramos cell transfectants. Expression of GFP-alone, GFP-GANP and GFP-ΔHATGconstructs were confirmed by blotting with the whole-cell lysate (WCL; input). Released mono- and poly- nucleosomes following MNase treatment were separated by agarose gel electrophoresis and detected by ethidium bromide (Et-Br). GANP presence in the chromatin fraction was detected using anti-GFP Ab. Histone acetylation was analysed by WB using anti-AcK, anti-H3 and anti-H3K9ac antibodies. Gel pictures are representatives from one of three sets of independent experiments with similar results. Figure 2: The histone acetylation activity of GANP modulates chromatin assembly and nucleosome organization. ( a ) The HAT domain of GANP (HAT G ) possesses histone acetylation activity. Recombinant GST-HAT G or GST-alone protein (100 ng) was incubated with histone H3 or H1 (1 μg) in the presence of acetyl-coenzyme A (10 μM). Acetylated histones H1 and H3 were analysed by WB. ( b ) MNase sensitivity assay for Ramos cell transfectants. Expression of GFP-alone, GFP-GANP and GFP-ΔHAT G constructs were confirmed by blotting with the whole-cell lysate (WCL; input). Released mono- and poly- nucleosomes following MNase treatment were separated by agarose gel electrophoresis and detected by ethidium bromide (Et-Br). GANP presence in the chromatin fraction was detected using anti-GFP Ab. Histone acetylation was analysed by WB using anti-AcK, anti-H3 and anti-H3K9ac antibodies. Gel pictures are representatives from one of three sets of independent experiments with similar results. Full size image Histone acetylation has been linked to dynamic changes in nucleosome organization that allow gene transcription upon activation [44] . We examined the effect of GANP on nucleosome assembly in Ramos B cells using an MNase sensitivity assay. Chromatin isolated from Ramos cells transfected with either GFP-GANP, or HAT-domain deleted GFP-GANP (GFP-ΔHAT G ) was treated with MNase and the resulting mono- and oligonucleosomal DNA was visualized using ethidium bromide ( Fig. 2b ). GFP-GANP overexpression markedly increased (about 4-fold) the amount of mononucleosomal and oligonucleosomal DNA released by MNase ( Fig. 2b , left and right), whereas the amount of released mononucleosomal DNA was not increased in GFP-ΔHAT G transfectants ( Fig. 2b , left). Regarding chromatin modification as the whole, GANP overexpression, but not GFP-ΔHAT G overexpression, causes a modest increase of histone H3 acetylation, as a distinct ~2-fold increase in acetylated H3K9 ( Fig. 2b , right). The data indicate that GANP modulates chromatin assembly and its role in nucleosome organization requires the HAT G domain with histone acetylation activity. We investigated the relevance of GANP for nucleosome positioning at the rearranged IgV-coding exons. The effect of GFP-GANP on positioning of nucleosomes at the rearranged VH4(DP63)JH6 locus in Ramos B cells was examined by a MNase resistance assay. Chromatin from GFP-GANP or GFP-alone transfectants was treated with MNase and the 15 overlapping DNA regions (100-bp each) covering the IgV-locus from the leader sequence were analysed by PCR ( Fig. 3a ). For transfectants with control GFP-alone, MNase resistance was observed at two specific sites of the rearranged IgV-locus: site A at the 5′-side (regions 4 and 5) covering the intron/exon junction and site B at the 3′-side site (regions 13, 14 and 15), situated close to the V-D-J joining site ( Fig. 3a ). Each site A and site B covers about 160 bp, suggesting that the coding IgV-region supports two stably assembled nucleosomes. GFP-GANP selectively lowered MNase resistance at site B but did not affect site A ( Fig. 3a ), indicating that GANP specifically disrupts assembly or stability of nucleosomes at the 3′-side of the IgV-locus. The effect of GANP on chromatin at site B depends on the HAT G domain, as the MNase-resistant profile of the GANP-transfectant lacking the HAT G domain (GFP-ΔHAT G ) is similar to the control transfectant ( Fig. 3a ). In the presence of transcription-elongation inhibitor actinomycin D (ActD) [45] , the MNase resistance of site B is significantly decreased, whereas site A is not affected ( Fig. 3b ), indicating that chromatin organization at the 3′-side of IgV undergoes changes during transcription. 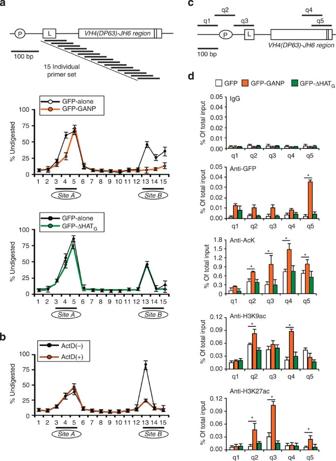Figure 3: GANP effects on nucleosome occupancy and histone modification at the rearranged Ig VH4(DP63)-JH4 locus. (a) Fifteen primer sets were designed to assay MNase resistance across the entire IgV-region (upper panel). Each bar shows the position of amplified region (100 bp). MNase resistance profile of VH4(DP63)-JH4 locus for GFP-GANP Ramos transfectants (middle panel) and GFP-ΔHATGtransfectants (lower panel). Values are the normalized amounts of the MNase-digested products to those of undigested samples. (b) Effect of ActD on MNase resistance profile VH4(DP63)-JH4 IgV-locus. Ramos cells were treated for 2 h with ActD (100 ng) followed by washing with PBS and incubation in the complete culture medium for 24 h. (c) GANP association to regions q1–q5 of the rearranged VH4(DP63)-JH6 locus and its effect on histone modifications. Scale is 100 bp. (d) ChIP-qPCR analysis of GFP-positive cells transfected with either GFP-alone (white columns), GFP-GANP (orange columns), or GFP-ΔHATG(green columns) using anti-GFP, anti-AcK, anti-H3K9ac and anti-H3K27ac antibodies. IgG was used as a negative control. Data represent mean±s.d. calculated from three (a,d) or two (b) independent experiments. *P<0.05 (two-tailed unpairedt-test). Figure 3: GANP effects on nucleosome occupancy and histone modification at the rearranged Ig VH4(DP63)-JH4 locus. ( a ) Fifteen primer sets were designed to assay MNase resistance across the entire IgV-region (upper panel). Each bar shows the position of amplified region (100 bp). MNase resistance profile of VH4(DP63)-JH4 locus for GFP-GANP Ramos transfectants (middle panel) and GFP-ΔHAT G transfectants (lower panel). Values are the normalized amounts of the MNase-digested products to those of undigested samples. ( b ) Effect of ActD on MNase resistance profile VH4(DP63)-JH4 IgV-locus. Ramos cells were treated for 2 h with ActD (100 ng) followed by washing with PBS and incubation in the complete culture medium for 24 h. ( c ) GANP association to regions q1–q5 of the rearranged VH4(DP63)-JH6 locus and its effect on histone modifications. Scale is 100 bp. ( d ) ChIP-qPCR analysis of GFP-positive cells transfected with either GFP-alone (white columns), GFP-GANP (orange columns), or GFP-ΔHAT G (green columns) using anti-GFP, anti-AcK, anti-H3K9ac and anti-H3K27ac antibodies. IgG was used as a negative control. Data represent mean±s.d. calculated from three ( a , d ) or two ( b ) independent experiments. * P <0.05 (two-tailed unpaired t -test). Full size image As nucleosomes are assembled at site A and site B of the rearranged IgV-locus ( Fig. 3a ), we examined GANP association with chromatin at the DNA regions surrounding the promoter and leader sequences of IgV H (regions q1, q2 and q3) and the regions at the V(D)J site (q4 and q5) ( Fig. 3c ). Ramos B cells were transfected with GFP-GANP, GFP-ΔHAT G or GFP-alone and subjected to ChIP assay by an anti-GFP Ab. GFP-GANP preferentially interacts with the q5 region of IgV H ( Fig. 3d ). GANP without the HAT G domain does not exhibit a preference in binding to the q5 region, indicating that GANP association with the q5 region is dependent on the HAT G domain ( Fig. 3d ). IgV-region chromatin modification regulated by GANP We examined epigenetic chromatin modifications at the VH4(DP63)JH6 locus ( Fig. 3c ) by comparing the levels of histone H3 acetylation at Lys9 (H3K9ac) and Lys27 (H3K27ac) in each of the q1 to q5 regions ( Fig. 3d ). Modified histone H3 is present at higher concentrations in regions q2 (H3K9ac) and q3 (H3K9ac and H3K27ac) that span the promoter and the immediate downstream leader sequence. GANP overexpression caused significant increases in H3K9ac and H3K27ac at the q2 region ( Fig. 3d , orange columns), H3K27ac at the q3 region, H3K9ac in the q4 region and H3K27ac at the q5 region. GANP appears to have no effect on chromatin modification at the promoter upstream region q1. The increase in histone H3 modifications at q2 to q5 regions is dependent on the HAT G domain ( Fig. 3d , green columns). Although GANP does not seem to possess histone-methyltransferase activity, GANP also increased the active transcription through chromatin modification with H3K4me3 presumably via regulation of methyltransferase activity ( Supplementary Table S1 and Supplementary Fig. S3 ). The preferential association of GANP with the q5 region and its ability to interact with and acetylate histone H1 and H3 ( Supplementary Table S2 and Fig. 2 ) suggest that GANP might be involved in regulation of acetylated H1K63ac and H3K27ac at q5 region. Interaction of GANP with the IgV transcription complex We investigated whether GANP interacts with the proteins involved in the transcription and targeting of AID to the IgV-locus. Co-IP analysis showed that RNA Pol-II and a transcription-stalling factor Spt5 associate with GANP in Ramos B cells ( Fig. 4a ). RNA Pol-II and Spt5 have been shown to interact with AID at IgV-loci [16] , [18] . The phosphorylation state of RNA Pol-II C-terminal domain (CTD) at Ser2 (pSer2) and Ser5 (pSer5) is often associated with changes in transcription stages [46] . Ser5 phosphorylation is required for the initiation of transcription at the promoter regions, whereas Ser2 phosphorylation is associated with mRNA elongation [46] . A ChIP assay with antibodies specific to pSer5 and pSer2 showed that GANP overexpression enhanced the binding of both pSer5 and pSer2 RNA Pol-II CTD to the q3–q5 region DNA of the IgV-region ( Fig. 4b ). GFP-ΔHAT G transfectants with a HAT G deletion, however, did not enhance RNA Pol-II binding to the IgV-region (q3-q5) ( Fig. 4b ), suggesting that the HAT G domain has an important role in facilitating RNA Pol-II access to the IgV-locus, presumably through histone modification. The concentrations of pSer5 and pSer2 are low and appeared unaffected by GANP at q1 region ( Fig. 4b ). 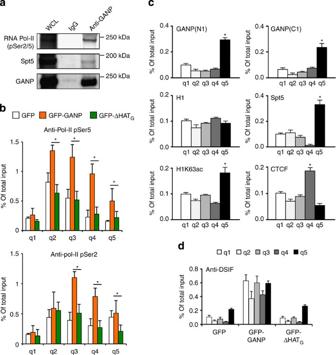Figure 4: GANP enhances recruitment of the transcription complex, transcription stalling factor Spt5 and DSIF (Spt4–Spt5 complex) to the IgV-locus. (a) Association of RNA Pol-II and Spt5 with GANP. Lysates from Ramos cells were IP using anti-GANP Ab. WB was carried out with anti-RNA Pol-II pSer2/5, anti-Spt5 or anti-GANP Ab. IgG was used as a negative control. Whole-cell lysate (WCL) is shown in the left. (b) ChIP-qPCR analysis of Ramos GFP-positive cells transfected with either GFP-alone (white columns), GFP-GANP (orange columns) or GFP-ΔHATG(green columns) for RNA Pol-II CTD phosphorylation at Ser5 and Ser2. (c) ChIP-qPCR assay for endogenous GANP, histone H1, H1K63ac, Spt5 and CTCF. Two different GANP antibodies, GANP (N1) and GANP (C1), anti-H1K63ac and anti-Spt5 were used to show preferred recruitment of GANP, H1K63ac and Spt5 to the q5 region. CTCF was found to associate preferentially at the q4 region. (d) ChIP-qPCR analysis of DSIF (Spt4 and Spt5). Data represent mean±s.d. calculated from three (b–d) or two (a) independent experiments. *P<0.05 (two-tailed unpairedt-test). Figure 4: GANP enhances recruitment of the transcription complex, transcription stalling factor Spt5 and DSIF (Spt4–Spt5 complex) to the IgV-locus. ( a ) Association of RNA Pol-II and Spt5 with GANP. Lysates from Ramos cells were IP using anti-GANP Ab. WB was carried out with anti-RNA Pol-II pSer2/5, anti-Spt5 or anti-GANP Ab. IgG was used as a negative control. Whole-cell lysate (WCL) is shown in the left. ( b ) ChIP-qPCR analysis of Ramos GFP-positive cells transfected with either GFP-alone (white columns), GFP-GANP (orange columns) or GFP-ΔHAT G (green columns) for RNA Pol-II CTD phosphorylation at Ser5 and Ser2. ( c ) ChIP-qPCR assay for endogenous GANP, histone H1, H1K63ac, Spt5 and CTCF. Two different GANP antibodies, GANP (N1) and GANP (C1), anti-H1K63ac and anti-Spt5 were used to show preferred recruitment of GANP, H1K63ac and Spt5 to the q5 region. CTCF was found to associate preferentially at the q4 region. ( d ) ChIP-qPCR analysis of DSIF (Spt4 and Spt5). Data represent mean±s.d. calculated from three ( b – d ) or two ( a ) independent experiments. * P <0.05 (two-tailed unpaired t -test). Full size image Preferential association of GANP with chromatin at the q5 region ( Fig. 3d ) was further examined for endogenous GANP in Ramos B cells. A ChIP assay using antibodies targeting either the N-terminus (N1) or C-terminus (C1) of GANP confirmed a preferential interaction of GANP to the q5 region of the IgV H ( Fig. 4c ). A ChIP assay was also used to examine the distribution of the histone H1, Spt5 and transcription pausing factor DSIF (Spt4-Spt5 complex) across the IgV-locus. The levels of unmodified histone H1 were similar in all q1 to q5 regions, but a significantly higher level of acetylated H1K63ac was observed at the q5 region ( Fig. 4c ). Similarly, the highest concentration of Spt5 was observed at the q5 region ( Fig. 4c ). In contrast to the enrichment of acetylated H1K63ac and Spt5 at the q5 region, the transcription insulator/repressor protein CTCF [47] exhibited preferential binding at the q4 region and lowest binding to the q5 region ( Fig. 4c ), suggesting that CTCF accesses the IgV-locus in a different manner. Full-length GANP enhanced the accessibility of DSIF at all regions with DSIF concentration distributed more or less evenly from the q1 to q5, suggesting that GANP overexpression promotes early recruitment of the elongation pausing factor DSIF to the transcription complex ( Fig. 4d ). GANP-mediated DSIF recruitment to IgV H is dependent on the HAT G domain ( Fig. 4d ). The effect of GANP on recruitment of DSIF to the IgV gene has an important implication for a possible mechanism of AID targeting. Perhaps, GANP-facilitated recruitment of the transcription factor DSIF causes stalling of RNA Pol-II at the IgV-region, providing AID access to the ssDNA within the transcription bubbles. Effects of GANP knockdown on IgV nucleosome occupancy We examined the physiological relevance of GANP by siRNA knockdown in Ramos B cells. Cy3 fluorescent-labelled siRNA (siGANP) targeting endogenous GANP severely reduced its expression in the sorted cells, but did not alter cellular levels of RNA Pol-II pSer2 and pSer5 ( Fig. 5a ). GANP knockdown caused a higher MNase resistance at both site A and site B of the IgV-locus ( Fig. 5b ). Consistent with GANP’s role in facilitating RNA Pol-II access to IgV ( Fig. 4b ), GANP downregulation led to a significant decrease in the levels of both pSer2 and pSer5 associated with each of the q1-q5 regions ( Fig. 5c ). Spt5 preferentially associates with the q5 region in control Ramos cells ( Figs 4c , 5c ), and it is noteworthy that there is a significant shift in the Spt5 positioning from the q5 to q3 region in GANP-knockdown cells ( Fig. 5c ). 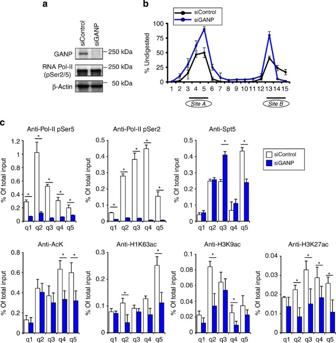Figure 5: Effects of downregulation of endogenous GANP on nucleosome occupancy and chromatin modification at Ig VH4(DP63)-JH4 locus. (a) Knockdown of GANP in Ramos B cells by fluorescent Cy3-labelled siRNA. GANP and RNA Pol-II expression in Cy3-positive sorted cells with control and GANP-targeted siRNA were examined by WB. (b) Analysis of nucleosome occupancy at the IgV-locus in control and GANP-knockdown Ramos B cells by the MNase resistance assay. (c) ChIP-qPCR analyses for pSer2, pSer5, Spt5 and modified histones H1 and H3 at q1 to q5 regions of the IgV-locus in GANP knockdown B cells. Data represent mean±s.d. calculated from two independent experiments. *P<0.05 (two-tailed unpairedt-test). Figure 5: Effects of downregulation of endogenous GANP on nucleosome occupancy and chromatin modification at Ig VH4(DP63)-JH4 locus. ( a ) Knockdown of GANP in Ramos B cells by fluorescent Cy3-labelled siRNA. GANP and RNA Pol-II expression in Cy3-positive sorted cells with control and GANP-targeted siRNA were examined by WB. ( b ) Analysis of nucleosome occupancy at the IgV-locus in control and GANP-knockdown Ramos B cells by the MNase resistance assay. ( c ) ChIP-qPCR analyses for pSer2, pSer5, Spt5 and modified histones H1 and H3 at q1 to q5 regions of the IgV-locus in GANP knockdown B cells. Data represent mean±s.d. calculated from two independent experiments. * P <0.05 (two-tailed unpaired t -test). Full size image The effects of GANP knockdown on the distribution of acetylated histones at the rearranged IgV-locus ( Fig. 5c ) are consistently opposite to those caused by GANP overexpression ( Figs 3d , 4b–d ). GANP knockdown and overexpression experiments also showed opposite effects on H3K9ac occupation at the regions q2 and q4 ( Figs 3d , 5c ). Together, both GANP knockdown ( Fig. 5 ) and GANP overexpression data ( Figs 3 , 4 ) suggest that GANP has an important role in epigenetic modification of chromatin at rearranged IgV-loci. Role of GANP in the IgV-region SHM We examined whether the transient increase of GANP expression can affect SHM at the IgV-locus. ChIP assay ( Fig. 6 and Supplementary Fig. S4 ) was used to capture IgV-regions that associate with H3K9ac, CTCF, GANP or AID. Mutational analysis of the captured IgV DNA showed that GANP exerted no effect on SHM of IgV associated with H3K9ac and CTCF. These IgV DNA exhibit low SHM with a frequency of 0.3–1.0 mutations per 10 3 bp ( Supplementary Fig. S3b,c ). GANP-bound IgV DNA showed similarly low mutation frequency (<0.3 mutations per 10 3 bp) [27] . However, GANP overexpression enhances SHM in AID-bound IgV DNA. The SHM frequency of AID-bound IgV increased 90% in the GFP-GANP transfectants (3.5 mutations per 10 3 bp) compared with that of GFP-alone transfectants (1.8 mutations per 10 3 bp) ( Supplementary Fig. S4a ). SHM in the AID-bound IgV DNA are about two-fold higher than IgV SHM in the input DNA, 1.72 mutations per 10 3 bp in GFP-GANP transfectants versus 0.85 mutations per 10 3 bp in GFP-control transfectants [27] . The higher SHM in AID-bound IgV compared with the input DNA, GANP-bound IgV and H3K9ac-bound IgV is consistent with the notion that SHM occurs only after recruitment of AID to the IgV-region, but not at the initial stage of GANP recruitment and chromatin modification. The analysis of base substitutions in AID-bound IgV DNA showed that majority of SHM mutations are G:C→A:T transitions, 36% G→A and 27% C→T in GFP-GANP transfectants, and 41% G→A and 6% C→T in GFP-control transfectants ( Supplementary Fig. S4a ). A comparison of SHM profiles of AID-bound IgV DNAs in GFP-GANP and GFP-control transfectants ( Fig. 5 ) showed that GANP overexpression augmented SHM over the entire rearranged IgV-region, in particular at nucleosome positioning site A and site B ( Fig. 6a ). 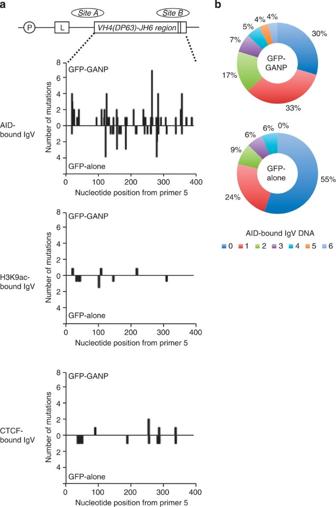Figure 6: AID targeting and SHM mutation distribution at the rearranged IgV-locus. (a) Mutation spectra of AID-bound IgV-region, H3K9ac-bound IgV-region and CTCF-bound IgV-region in GFP-alone and GFP-GANP Ramos cell transfectants. DNAs isolated from anti-AID, anti-H3K9Ac and anti-CTCF Ab IP samples were subjected to sequencing analysis. SHM mutation profiles of IgV DNA starting from the primer 5 (DP63-05S) were shown. (b) Pie charts showing the distribution of numbers of mutations per a sequenced clone for AID-bound IgV-region from GFP-GANP and GFP-alone transfectants. Data are from one of three independent experiments with similar results. Figure 6: AID targeting and SHM mutation distribution at the rearranged IgV-locus. ( a ) Mutation spectra of AID-bound IgV-region, H3K9ac-bound IgV-region and CTCF-bound IgV-region in GFP-alone and GFP-GANP Ramos cell transfectants. DNAs isolated from anti-AID, anti-H3K9Ac and anti-CTCF Ab IP samples were subjected to sequencing analysis. SHM mutation profiles of IgV DNA starting from the primer 5 (DP63-05S) were shown. ( b ) Pie charts showing the distribution of numbers of mutations per a sequenced clone for AID-bound IgV-region from GFP-GANP and GFP-alone transfectants. Data are from one of three independent experiments with similar results. Full size image GANP enhances AID-accessibility at IgV-regions in GC B cell We examined whether GANP affects the chromatin occupancy of AID at the rearranged IgV-locus in B cells during the immune response ( Fig. 7 ). Mice with a conditional Ganp -knockout in CD19 B cells ( CD19Cre/Ganp F/F ), the control floxed/floxed C57BL/6 ( Ganp F/F ), the Ganp -gene transgenic B cells ( Ganp Tg ) and the control C57BL/6 ( WT ) were immunized with nitrophenyl-chicken γ-globulin (NP-CGG) in alum conjugates for 14 days and spleen GC B-cells were sorted by using mature GC B cell markers of B220, GL-7 and Fas ( Supplementary Fig. S5 ). The mutant mice showed no measurable difference in Aicda transcription, but the transcription of the IgV H 186.2-region was significantly enhanced in GC B cells with higher GANP expression from ganp Tg mice ( Fig. 7a ). In contrast, GC B cells from Ganp -deficient ( CD19-Cre/Ganp F/F ) mice showed significantly lower amounts of IgV H 186.2-region transcripts ( Fig. 7a ). The chromatin occupancy was measured by a ChIP assay using a primer combination that amplifies the IgV H 186.2-locus encoding the NP-binding IgV heavy chain. GANP overexpression showed a marked increase of AID-binding to the IgV H 186.2-region, and particularly to the region that displayed the increased AID binding ( Fig. 7b ). Reciprocally, Ganp deficiency significantly decreased AID-binding to the IgV H 186.2-region ( Fig. 7c ). The results indicated that GANP indeed helps AID to access the IgV-region in GC B cells. 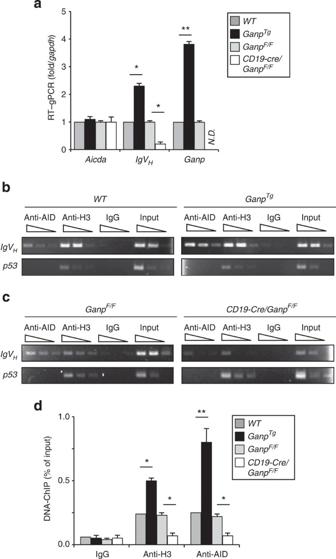Figure 7: GANP enhances the accessibility of AID to IgVH-region DNA in mouse GC B cells. (a) RT–qPCR analysis ofGanp,AicdaandIgVHtranscripts in GC B cells fromWT,GanpTg,GanpF/FandCD19-Cre/GanpF/F(n=3 mice per genotype). (b) ChIP analysis of GC B cells ofWTandGanpTg. Input and ChIP samples were serially diluted 1:3 (wedge) and various genomic DNA sequences (left margin) were amplified with specific primers and were detected by ethidium bromide (Et-Br) staining. Anti-histone H3 (H3) Ab was used as a positive control. (c) ChIP analysis in GC B cells of the controlGanpF/FandGanp-deficientCD19-Cre/GanpF/F, as inb. (d) ChIP-qPCR analysis of GC B cells fromWT,GanpTg,GanpF/FandCD19-Cre/GanpF/F. ChIP was amplified by qPCR with specific primers. Data (a,d) represent mean±s.d. calculated from three independent experiments *P<0.05 and **P<0.01 (two-tailed unpairedt-test). Figure 7: GANP enhances the accessibility of AID to IgV H -region DNA in mouse GC B cells. ( a ) RT–qPCR analysis of Ganp , Aicda and IgV H transcripts in GC B cells from WT , Ganp Tg , Ganp F/F and CD19-Cre/Ganp F/F ( n =3 mice per genotype). ( b ) ChIP analysis of GC B cells of WT and Ganp Tg . Input and ChIP samples were serially diluted 1:3 (wedge) and various genomic DNA sequences (left margin) were amplified with specific primers and were detected by ethidium bromide (Et-Br) staining. Anti-histone H3 (H3) Ab was used as a positive control. ( c ) ChIP analysis in GC B cells of the control Ganp F/F and Ganp -deficient CD19-Cre/Ganp F/F , as in b . ( d ) ChIP-qPCR analysis of GC B cells from WT , Ganp Tg , Ganp F/F and CD19-Cre/Ganp F/F . ChIP was amplified by qPCR with specific primers. Data ( a , d ) represent mean±s.d. calculated from three independent experiments * P <0.05 and ** P <0.01 (two-tailed unpaired t -test). Full size image GANP has been characterized as a component of the mRNA export TREX-2-complex based on a homology comparison with yeast Sac3 (refs 35 , 39 ). In mammals, the nascent mRNAs need to undergo extensive processing, which includes 5′-capping, splicing and 3′-end polyadenylation to become mature mRNAs. Only properly spliced and mature RNAs can be assembled into a RNP nuclear export complex, which is then exported through the nuclear pores to the cytoplasm [48] . 2DICAL analysis revealed GANP interactions with proteins involved in mRNA processing and splicing factors and Nup proteins ( Supplementary Table S1 and Supplementary Fig. S2b ). These results are consistent with the role of GANP in nuclear export of mRNA (ref. 35 ). The increase of GANP in GC B cells during the immune response [28] seems to have a distinct role through selective interaction with the rearranged IgV-loci and perhaps in the RNP complex undergoing the unique process of RNA metabolism with nuclear cytidine deaminases in higher eukaryote cells. This may imply a role for GANP distinct from that of the prototype Sac3 (refs 32 , 33 ). GANP appears to enhance chromatin modifications and it might have a significant role at the initial step of chromatin modification at the rearranged IgV loci. Particularly, the linker histone H1 was found to be associated with GANP by 2DICAL analysis ( Supplementary Table S2 ). Modifications of the linker histone lead to the relaxation of the compact chromatin structure assembled with core histones. ChIP analysis showed that the acetylated histone H1 (H1K63ac) is found preferentially at the q5 region of the rearranged IgV-locus in B cells ( Fig. 4c ). A similar high concentration of endogenous GANP at the q5 region suggests that HAT G domain of GANP is necessary to acetylate histone H1 at this region. The observed increase in acetylated histone H1, which unfolds the chromatin at the q5 region, is consistent with an increase in mononucleosome release ( Fig. 2b ) and a higher MNase sensitivity at the 3′-side site B of IgV H in the presence of overexpressed GANP ( Fig. 3b ). The involvement of GANP in chromatin modification at the IgV-locus is further supported by experiments in which GANP is downregulated by siRNA. GANP knockdown ( Fig. 5 ) and GANP overexpression ( Figs 3 , 4 ) lead to opposing effects on the levels of modified histones H1K63ac, H3K9ac and H3K27ac at specific regions within the IgV-locus. Although GANP prefers binding to the 3′-side of the IgV-locus (region q5) and exerts its strongest effects on chromatin modification and nucleosome assembly at site B , it also exerts significant effects on chromatin at other IgV-regions. For example, cells in which GANP is downregulated by siRNA ( Fig. 5 ) exhibit higher resistance to MNase at both sites A and B . Changes in GANP expression also significantly affect the levels of modified histone H3 (H3K9ac and H3K27ac) at the promoter and leader sequences (regions q2 and q3) of the IgV-locus ( Figs 3 , 4 , 5 ). Transcription at the rearranged IgV-locus is regulated by cooperation of the B cell specific transcription factors operating at the 5′-promoter region and the intronic enhancer region. The chromatin at the Ig-locus inevitably undergoes alterations, transforming from the germ line structure to the functionally rearranged V H -D H -J H region by V(D)J recombination, which randomly joins V, D and J segments and cleaves out the long intervening V, D and J genomic segments. The altered chromatin folding along with extensive histone modification opens up the chromatin structure to allow access by RNA Pol-II and various transcription factors. Indeed, during V H -D H -J H recombination, the RAG-associated complex creates recombination centres containing increased concentration of H3K9ac, H3K4me3 and RNA Pol-II (refs 49 , 50 ). In B cells, GANP is preferentially associated with the 3′-end of the rearranged V H -D H -J H exons ( Fig. 4c ). In the absence of exogenously expressed GANP, the transcription stall factor DSIF (Spt4–Spt5 complex) is also present at a highest concentration at the same site ( Fig. 4c ). Importantly, GANP overexpression significantly enhances DSIF recruitment to all q1–q5 regions spanning the entire IgV H from the promoter to the 3′-end of V-D-J junction ( Fig. 4d ). The uniform distribution of DSIF across these regions ( Fig. 4d ) suggests that GANP promotes early recruitment of DSIF to the IgV transcription complex. Early recruitment of DSIF at the promoter 5′-site of IgV may ensure the efficient induction of RNA Pol-II stalling throughout the entire IgV-coding region covering complementarity-determining regions 1 and 2. How GANP regulates early recruitment of DSIF to the IgV-locus is not yet clear. GANP interacts with Spt5 ( Fig. 4a ), and as both proteins associate preferentially with q5 ( Figs 4c , 5c ), we suggest that GANP might be involved in the recruitment of Spt5 to q5. Alternatively, increased transcription of IgV-locus might also be responsible for recruitment of Spt5 or an Spt5-loading factor such as PAF1 (ref. 19 ). The role of Spt5 in transcription pausing and maintenance of R-loop has recently been proposed at the S-region of the Ig gene during class switch recombination [15] , [16] . Similar to the RNA Pol-II stalled model for increased AID access to the S-region, we propose that GANP promotes early recruitment of DSIF, enabling frequent pausing of the transcription complex along the IgV-locus. GANP is associated with the site B nucleosome position at the IgV-locus, the q5 region, and through GANP-AID protein–protein interaction [27] , recruits AID to the nearby stalled transcription bubbles at IgV ( Fig. 8 ). Within the stalled bubbles, AID can access deoxycytidine on exposed ssDNA of the non-transcribed strand, or through interaction with an exosome complex to access the transcribed strand [15] . 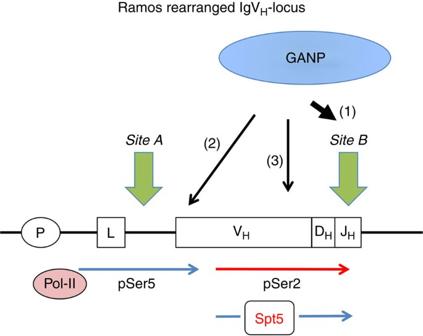Figure 8: A model of GANP-mediated AID targeting for SHM at the IgV-loci. GANP associates with histones H1 and H3, the IgV transcription–elongation complex, and the transcription stall factor Spt5 in Ramos B cells. The rearranged IgV-locus supports two stably assembled nucleosomes atsite Aandsite B. GANP is involved in chromatin remodelling at the IgV-locus through its HAT domain and causes destabilization of nucleosome assembly atsite B(1). Chromatin remodelled IgV provides increased access for both pSer5 and pSer2 forms of RNA Pol-II leading to an increase in IgV transcription (2). GANP facilitates early recruitment of the DSIF transcription stalling complex (Spt4–Spt5) to the IgV-coding region, causing frequent stalling of transcription bubbles, which provide ssDNA substrates for AID-targeting (3). Figure 8: A model of GANP-mediated AID targeting for SHM at the IgV-loci. GANP associates with histones H1 and H3, the IgV transcription–elongation complex, and the transcription stall factor Spt5 in Ramos B cells. The rearranged IgV-locus supports two stably assembled nucleosomes at site A and site B . GANP is involved in chromatin remodelling at the IgV-locus through its HAT domain and causes destabilization of nucleosome assembly at site B (1). Chromatin remodelled IgV provides increased access for both pSer5 and pSer2 forms of RNA Pol-II leading to an increase in IgV transcription (2). GANP facilitates early recruitment of the DSIF transcription stalling complex (Spt4–Spt5) to the IgV-coding region, causing frequent stalling of transcription bubbles, which provide ssDNA substrates for AID-targeting (3). Full size image Chromatin modification is probably essential for subsequent molecular steps for augmenting SHM in GC B cells. The 3′ nucleosome positioning site ( site B ) of the rearranged IgV exons may serve as an anchor site for recruitment of GANP, transcription factor Spt5 and other proteins involved in AID targeting. An increase in GANP expression promotes histone H3 modifications at IgV covering all regions from the promoter to the 3′-side ( Fig. 3d ). GANP-mediated chromatin remodelling at IgV likely provides better access for RNA Pol-II, reflected by increases in both phosphorylated pSer5 and pSer2 forms ( Fig. 4a ). The early recruitment of DSIF to the IgV transcription complex results in an increased concentration of stalled transcription bubbles throughout the IgV-regions to which AID is targeted. Once AID is bound to the ssDNA substrate within the bubbles, AID may stay associated with DNA and travel along with an elongating transcription complex across the IgV-region as proposed in a random walk model in an in vitro study [51] . The altered chromatin modification by GANP might affect AID access to the IgV locus in GC B cells. The chromatin occupancy of AID at the IgV-locus was significantly decreased in Ganp -deficient B cells by conditional gene targeting ( Fig. 7c ) and reciprocally augmented by GANP overexpression in Ganp Tg mice ( Fig. 7b ). All of these observations taken together suggest that GANP is involved at an early stage of Ig transcription by assisting the modification of histones and by interaction with nucleosomes at the 3′-side of the rearranged IgV exon. GANP-mediated chromatin modification appears to facilitate the early recruitment of the transcription stalling factor DSIF, leading to a high concentration of stalling transcription bubbles within the entire IgV-coding region. Through its direct interaction, GANP then helps recruitment of AID to the stalled bubbles to initiate SHM, an essential process for affinity-maturation of antibodies against Ags during immune responses. Cell culture Cells were maintained in DMEM (for 293 T) and RPMI-1640 medium (for Ramos) supplemented with 10% heat-inactivated FBS (Invitrogen). Antibodies Antibodies to AID (L7E7 and 30F12; Cell Signalling Technology (CST)), GFP (ab290; Abcam), FLAG (M2; Sigma-Aldrich), mouse IgG (sc-2025; Santa Cruz), rabbit IgG (sc-2027; Santa Cruz), pan-AcK (no. 9441; CST), H3 (no. 4620, CST), H3K9ac (Y28, Millipore), H3K4me3 (no. 9751; CST), H3K27ac (no. 4353; CST), CTCF (no. 3418; CST), H1 (ab71594; Abcam), H1K63ac (ab32145; Abcam), RNA Pol-II (ab817; Abcam), pSer2 (ab5095; Abcam), pSer5 (ab5131; Abcam), and pSer2/5 (no. 4735; CST) of RNA Pol-II CTD, DSIF (611106; BD Biosciences), Spt5 (sc-28678; Santa Cruz), GANP (HPA021527; Sigma-Aldrich, 11054-AP; ProteinTech; sc-83297; Santa Cruz) were used. The purified splenic B cells were stained with antibodies to GL-7, CD45R/B220 and CD95/Fas (BD Biosciences), each conjugated to a different fluorochrome. Preparation of nuclear extract Ramos cells (5 × 10 7 cells) were resuspended in Buffer A (10 mM Tris-HCl pH 7.9, 1 mM EDTA, 5 mM DTT) on ice for 20 min and lysed by Dounce homogenizer ‘loose’ pestle (Ikemoto, Japan) (eight strokes). Nuclei were harvested by centrifuged at 4,000 r.p.m. for 10 min and resuspended in buffer B (50 mM Tris-HCl pH 7.9, 10 mM MgCl 2 , 2 mM DTT, 25% (g/v) sucrose, 50% (v/v) glycerol). The nuclei were lysed by Dounce homogenizer pestle (eight strokes) followed by dropwise addition of ammonium sulphate and gentle stirring for 30 min. Following centrifugation at 45,000 r.p.m. (60T1 rotor) for 3 h, the supernatant was collected and ammonium sulphate (0.33 g ml −1 of solution) was added to precipitate nuclear proteins. The nuclear proteins were collected by centrifugation at 15,000 r.p.m. for 20 min and resuspended in buffer C (25 mM HEPES pH 7.9, 100 mM KCl, 12 mM MgCl 2 , 0.5 mM EDTA, 2 mM DTT, 17% (v/v) glycerol) followed by extensive dialysis against Buffer C to remove excess salt. Nuclear proteins were stored in small aliquots at −80 °C. All steps were carried out at 4 °C. 2DICAL analysis 2DICAL analysis was performed as previously [40] , [41] . Briefly, the Ramos nuclear extract was mixed with 5 μg of anti-GANP Ab in 1 ml volume for overnight, then the complex was precipitated with Dynabeads Protein A (VERITAS). Precipitants were washed six times with detergent-free RIPA buffer (50 mM Tris-HCl pH 7.5, 150 mM NaCl, 1 mM EDTA, 0.05% (g/v) of SDS) supplemented with protease inhibitors. The beads were suspended in 1% (g/v) sodium deoxycholate and then boiled. The eluate was subjected to the proteomics analysis. Plasmid construct GANP mutant deleted at the HAT-region was constructed by joining of the two truncated (N-half and C-half) ganp cDNAs prepared separately by the inverted PCR. Primers used are as follows: 0700-S; 5′-GGGTCGACATGCACCCGGTGAACCCCTTCG-3′ 1400-S; 5′-ACCAGACGCAGCAAGAAGCT-3′ 2800-S; 5′-GAATCGGTCGGCATTCTTGG-3′ ΔHAT-N (H-N-AS); 5′-GGGGTCGACCTCTGGTGAGTTCCAGTG-3′ ΔHAT-C (H-C-S); 5′-GGGCTCGAGCACGTTCCCTCGTCATGG-3′ For GST-HAT G construct, the HAT-region was amplified with 5′-GGGACTAGTGAGCACCTGGCCTGGCTGAA-3′ and 5′-GGGCTCGAGCTACGACAAAGGAACATCATATT-3′ primers and generated in pET41 vector. All constructs were verified by sequencing on both strands. Purification of recombinant proteins Recombinant GST, and GST-HAT G proteins were purified from a BL21(DE3) E. coli strain transformed with pET41 vector. GST-fusion proteins were dialyzed in 20 mM Tris-HCl pH 8.0, 50 mM NaCl, 1 mM DTT, 10% (v/v) glycerol and stored at −80 °C. Purification of crude histones Core histones were purified from Ramos cells by using histone purification kit (Active Motif) according to the manufacturer’s protocol. In vitro histone acetylation assay Non-isotopic in vitro histone acetylation assay was carried out with a minor modification [52] . Briefly, recombinant GST or GST-HAT G protein (100 ng each) was incubated with histone H3 or H1 (1 μg) in the presence of 10 μM acetyl-coenzyme A (Sigma) in 50 μl reaction buffer 50 mM Tris-HCl pH 8.0, 10% (v/v) glycerol, 10 mM butyric acid, 0.1 mM EDTA, 1 mM DTT and 1 mM PMSF at 30 °C on a rotating platform. At 5, 10, 15, 30, 45 and 60 min, aliquots were withdrawn and quenched with Laemmli buffer. Acetylated histones H1 and H3 were separated by SDS–PAGE and analysed by WB using anti-AcK Ab. Transfection and knockdown Transfection was performed as previously [27] . Knockdown experiment was carried as follows: 293 T plated in a 10 cm-dish with 1 × 10 6 cells was transfected in OPTI-MEM GlutaMAX medium with 2 nM of small interfering RNA (siRNA, Sigma, Supplementary Table S3 ) using lipofectamine RNAiMAX (Invitrogen) transfection reagent. For B cell knockdown experiment, cells were transfected with 2 μM of fluorescent Cy3-labelled control or GANP-targeted siRNA using the Amaxa Nucleofection Kit V (program O-06) and Cy3-positive cells were sorted. Preparation of native chromatins and nucleosomes Cells were lysed in TEB buffer (PBS containing 0.05% (v/v) TritonX-100, 2 mM PMSF, 5 mM sodium butyrate, and the protease inhibitor cocktail (Nacalai Tesque)). The nuclei were obtained with gentle stirring on ice. After the pellet was washed twice with MNase digestion buffer (0.32 M sucrose, 50 mM Tris-HCl pH 7.5, 4 mM MgCl 2 , 1 mM CaCl 2 , 0.1 mM PMSF and 5 mM sodium butyrate), mononucleosomes were prepared by digestion with 10 U of MNase at 37 °C for 5 min. Cell sorting GFP + (both GFP-alone, GFP-GANP and GFP-ΔHAT G ) populations of Ramos B cells or B220 + GL-7 + Fas + population of GC B cells from Ag-immunized mice were purified by FACSAria cell sorter system (BD Biosciences). Nucleosome positioning assay Crude nuclear extracts were treated with or without 10 U of MNase to digest the nucleosomes. After incubation at 37 °C for 30 min, the genomic DNA was purified. The nucleosome positions recognized by the antibodies were determined by the specific amplification of the DNA region with 15 primer sets ( Supplementary Table S3 ) by qPCR and shown as the ratio of the amount of digested/undigested DNAs. Ramos cells were treated with 0.1 μg of ActD (Nacalai Tesque) for 120 min. ChIP and qPCR ChIP assay was performed as reported previously [27] . The ChIP products were measured by using MESA BLUE qPCR Master Mix Plus (Eurogentec) on the Applied Biosystems 7500 Fast (Applied Biosystems) with specific primers ( Supplementary Table S3 ). Total RNA was isolated using an RNeasy Micro Kit (QIAGEN GmbH, Germany) and cDNA was generated using a SuperScript III First-Strand Synthesis System (Invitrogen, Carlsbad, CA) according to the manufacturers’ protocols. Real-time qPCR was performed using Applied Biosystems 7500 (Applied Biosystems) and THUNDERBIRD SYBR qPCR Mix (TOYOBO) or TaqMan probe ( Supplementary Table S3 ) and Universal PCR Master Mix, with No AmpErase UNG (Applied Biosystems). The transcript of each gene was calculated by a standard curve method and normalized to the expression of gapdh . Sequence analysis of the IgV H gene The rearranged IgV H of Ramos cells was amplified with the primer set of 5′-TGTTCACAGGGGTCCTGTCCCAGGTGCAGC-3′ and 5′-CTGAGGAGACGGTGACCGTGGTCCCT-3′. The V H 186.2 allele was amplified with the primer set of 5′-TTCTTGGCAGCAACAGCTACAGGTAAGG-3′, and 5′-GCAGGCTTGAGGTCTGGACATATACATG-3′. The PCR products by PrimeSTAR HS polymerase (Takara Bio Inc.) were ligated into the pCR4 Zero Blunt TOPO sequencing vector (Invitrogen) and then sequenced using ABI3130 Genetic Analyser with a BigDye Terminator (Applied Biosystems). Mice Ganp Tg (C57BL/6 J-TgN[GANP]meg), WT , Ganp F/F (Mcm3ap tm1Imku /Mcm3ap tm1Imku ) and CD19-Cre/Ganp F/F (Cd19 tm1(cre)Cgn /Cd19+ X Mcm3ap tm1Imku /Mcm3ap tm1Imku ) mice were used. Isolation of GC B cells was described previously [27] . All mice were maintained in the Centre for Animal Resources and Development, Kumamoto University. All studies and procedures were approved by the Kumamoto University Animal Care and Use Committee. Statistical analysis The statistical significance of differences between two groups was examined by an unpaired two-tailed Student’s t -test. P- values of less than 0.05 or 0.01 were considered significant and very significant, respectively. How to cite this article: Singh, S. K. et al . GANP regulates recruitment of AID to immunoglobulin variable regions by modulating transcription and nucleosome occupancy. Nat. Commun. 4:1830 doi: 10.1038/ncomms2823 (2013).